Atomically precise nanoclusters with reversible isomeric transformation for rotary nanomotors 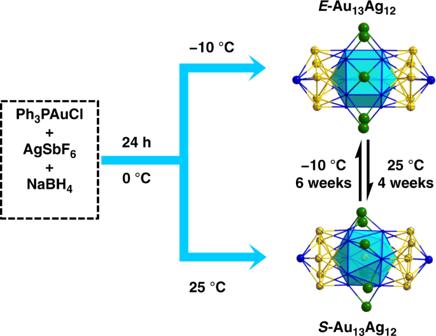Fig. 1: Two isomers of the [Au13Ag12(PPh3)10Cl8]+(SbF6)ˉ nanocluster with thermally responsive transformation (h = hour). E-eclipsed configuration,S-staggered configuration. Color code: Au: yellow; Ag: blue; Cl: green (C, H, P, and some Cl are omitted for clarity). Thermal-stimuli responsive nanomaterials hold great promise in designing multifunctional intelligent devices for a wide range of applications. In this work, a reversible isomeric transformation in an atomically precise nanocluster is reported. We show that biicosahedral [Au 13 Ag 12 (PPh 3 ) 10 Cl 8 ]SbF 6 nanoclusters composed of two icosahedral Au 7 Ag 6 units by sharing one common Au vertex can produce two temperature-responsive conformational isomers with complete reversibility, which forms the basis of a rotary nanomotor driven by temperature. Differential scanning calorimetry analysis on the reversible isomeric transformation demonstrates that the Gibbs free energy is the driving force for the transformation. This work offers a strategy for rational design and development of atomically precise nanomaterials via ligand tailoring and alloy engineering for a reversible stimuli-response behavior required for intelligent devices. The two temperature-driven, mutually convertible isomers of the nanoclusters open up an avenue to employ ultra-small nanoclusters (1 nm) for the design of thermal sensors and intelligent catalysts. Stimuli-responsive materials are at the forefront of technological innovations to fabricate the next-generation devices with “intelligent” performance [1] , [2] , [3] . To meet the self-activation and -deactivation functionality requirements for smart materials, the stimuli-responsive behavior should be reversible. This can be satisfied by utilization of precise structural and phase transitions [4] , [5] , [6] , [7] , [8] . In particular, reversible conformational isomerism, a fundamental concept in molecular sciences that is commonly observed in organic molecules, offers a unique platform to prepare rotary motors at the nanoscale with atomistic precision. Despite recent advances in controllable synthesis and structure determination of atomically precise nanoclusters [9] , [10] , [11] , [12] , [13] , [14] , [15] , [16] , [17] , [18] , the concept of reversible conformational isomerization for metal nanoclusters has not yet been explored. To date, irreversible structural isomerization of atomically precise nanoclusters has been reported in a few cases [19] , [20] , [21] , [22] , [23] , [24] . One case pertains to Au 42 (TBBT) 26 (TBBT = 4-tert-butylbenzenethiolate) in the form of fcc and non-fcc frameworks that were synthesized via two different procedures [19] . However, the two isomeric structures of Au 42 are “static” and cannot be reversibly transformed [19] . The same is true to the clusters prepared by Teo et al. [20] , [21] , [22] , [23] . One directional structural conversion from metastable Au 38 (SC 2 H 4 Ph) 24 to thermodynamically stable biicosahedral Au 38 (SC 2 H 4 Ph) 24 was reported to occur under thermal conditions, but unfortunately the reverse transformation could not occur [24] . Finally, while reversible transformation between Au 28 (SC 6 H 11 ) 20 and Au 28 (SPhC 4 H 9 ) 20 nanoclusters was realized by Chen et al., this case involves different surface-protecting ligands (-SC 6 H 11 vs. -SC 4 H 9 ), so it does not strictly meet the definition of isomeric transformation [25] and cannot be utilized for construction of nanomotors. Therefore, breakthroughs are still needed to precisely modulate the bonding structure of ultra-small nanoparticles to make their frameworks flexible for a facile molecular rotary nanomotor. Herein, we report the discovery of a stimuli-responsive nanocluster that shows reversible conformational isomerism. The [Au 13 Ag 12 (PPh 3 ) 10 Cl 8 ] + (SbF 6 )ˉ nanocluster, hereafter abbreviated as Au 13 Ag 12 , presents two isomeric forms that can be selectively obtained by simply controlling the temperature (Fig. 1 ), hence forming the basis of a rotary nanomotor controlled by temperature. Through a combined approach of experiments, we have investigated the structure of the nanocluster and its stimuli-responsive isomerization. The isomers possess distinct optical properties, which can be utilized for advancing intelligent sensors, catalysts, and controlled drug release in biomedical applications. Fig. 1: Two isomers of the [Au 13 Ag 12 (PPh 3 ) 10 Cl 8 ] + (SbF 6 )ˉ nanocluster with thermally responsive transformation (h = hour). E- eclipsed configuration, S- staggered configuration. Color code: Au: yellow; Ag: blue; Cl: green (C, H, P, and some Cl are omitted for clarity). Full size image Synthesis and characterization of Au 13 Ag 12 isomers The Au 13 Ag 12 nanocluster was synthesized by reduction of a mixed solution of Ph 3 PAuCl and AgSbF 6 using NaBH 4 in an ice bath (see Supplementary Methods). The nanoclusters were analyzed by electrospray ionization mass spectrometry (ESI-MS) in a positive mode. A weak mass peak at m / z = 6762.10 and an intense one at m / z = 3362.56 were observed in the mass spectrum (Fig. 2a ), with the spacing of their isotope patterns being 1 and 0.5 (Fig. 2a , inset), hence, 1+ and 2+ charges, respectively. The two mass peaks correspond to [Au 13 Ag 12 (PPh 3 ) 10 Cl 8 ] + (theoretical m / z : 6761.46 Da, deviation: 0.62 Da) and [Au 13 Ag 12 (PPh 3 ) 10 Cl 7 ] 2+ (theoretical m / z : 3363.00 Da, deviation: −0.44 Da), respectively, with the latter (2+ ion) being formed via loss of a Cl − from the intact 1+ cluster during the ESI-MS analysis. X-ray crystallographic analysis (vide infra) confirmed homogeneous [Au 13 Ag 12 (PPh 3 ) 10 Cl 8 ] + , with no observation of [Au 13 Ag 12 (PPh 3 ) 10 Cl 7 ] 2+ . It is worth noting that loss of a Cl − ligand often occurs in ESI-MS analysis [26] . Therefore, the molecular formula of the synthesized nanoclusters is [Au 13 Ag 12 (PPh 3 ) 10 Cl 8 ] + , and the product is highly pure. Fig. 2: Characterization of the Au 13 Ag 12 nanoclusters. a Positive-mode ESI mass spectrum of the as-synthesized Au 13 Ag 12 nanocluster. (M = Au 13 Ag 12 (PPh 3 ) 10 Cl 8 ) b Thin-layer chromatography separation of the Au 13 Ag 12 using CH 2 Cl 2 /CH 3 OH (2:1, v/v) as an eluent. c 31 P NMR spectra of the S -Au 13 Ag 12 and E -Au 13 Ag 12 in CD 2 Cl 2 . Full size image Surprisingly, two species were identified in the Au 13 Ag 12 product by thin-layer chromatography (TLC) with CH 2 Cl 2 /CH 3 OH (2:1, v/v) as the eluent [27] . The two distinct bands (Fig. 2b ) indicate two isomers of Au 13 Ag 12 since they share the same composition, hereafter denoted as E - and S -Au 13 Ag 12 (vide infra). The bands were cut out and extracted with CH 2 Cl 2 , and their optical spectra indeed show different profiles of the two isomers of Au 13 Ag 12 (see Supplementary Fig. 1 ). The ultraviolet–visible (UV-vis) spectrum of the mixed isomers exhibit peaks at 324, 361, 420, 500, and 656 nm. After TLC separation, the E -Au 13 Ag 12 nanocluster shows three peaks at 361, 418, and 497 nm, whereas the S -Au 13 Ag 12 isomer shows four peaks at 330, 423, 510, and 657 nm. The energy gaps of the S - and E -Au 13 Ag 12 isomers are 1.72 and 2.17 eV, respectively (see Supplementary Fig. 1 , inset). Interestingly, the pure S - and E -Au 13 Ag 12 isomers show different 31 P nuclear magnetic resonance (NMR) signals: 54.80 ppm for E -Au 13 Ag 12 and 57.36 ppm for S -Au 13 Ag 12 using Au(PPh 3 )Cl ( 31 P NMR: 33.13 ppm) as the internal reference (Fig. 2c and see Supplementary Fig. 2 ). It demonstrates that the E -Au 13 Ag 12 and S -Au 13 Ag 12 nanoclusters have different structures (vide infra). 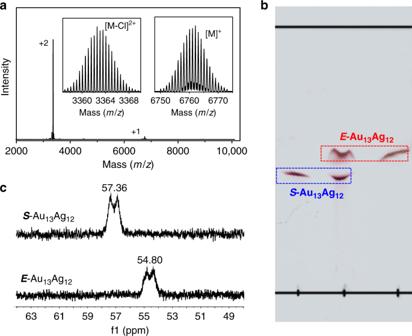Fig. 2: Characterization of the Au13Ag12nanoclusters. aPositive-mode ESI mass spectrum of the as-synthesized Au13Ag12nanocluster. (M = Au13Ag12(PPh3)10Cl8)bThin-layer chromatography separation of the Au13Ag12using CH2Cl2/CH3OH (2:1, v/v) as an eluent.c31P NMR spectra of theS-Au13Ag12andE-Au13Ag12in CD2Cl2. Crystal structures Furthermore, we found that keeping a fresh solution of the Au 13 Ag 12 nanocluster containing both isomers at 25 °C for 4 weeks led to a solution containing only the S -Au 13 Ag 12 isomer. In contrast, under −10 °C the same isomeric mixture completely transforms to the E -Au 13 Ag 12 isomer after 6 weeks. Crystallizations of the S -Au 13 Ag 12 and E -Au 13 Ag 12 isomers were performed via a vapor diffusion method, followed by X-ray diffraction analysis. The total structures of S -Au 13 Ag 12 and E -Au 13 Ag 12 are displayed in Supplementary Figs. 3 and 4 . For the core frameworks, each isomer is composed of two icosahedral Au 7 Ag 6 units fused together by sharing a common vertex of Au (Fig. 3a ). The two Au 5 pentagons at the ends of the rod are ligated by ten phosphine ligands. Two Cl ligands bind with two apical Ag atoms. Six Cl ligands bridge the two icosahedra via bonding with 10 equatorial Ag atoms (see Supplementary Fig. 5 ). Fig. 3: Configuration of the Au 13 Ag 12 nanocluster. a , b Two icosahedral Au 7 Ag 6 units share one common vertex of Au to form the Au 13 Ag 12 nanocluster. c Metal configuration of E -isomer. d Metal configuration of S -isomer. Color code: Au: yellow; Ag: blue. Other atoms are omitted for clarity. Full size image The central Au atom (enlarged in Fig. 3b ) connects the two Au 7 Ag 6 icosahedra and serves as the pivot for the rotamerization of the metal configuration of the Au 13 Ag 12 . At −10 °C, the two Au 7 Ag 6 units are in an eclipsed ( E ) configuration with D 5h symmetry (i.e., E -Au 13 Ag 12 , Fig. 3c ), whereas at 25 °C the two Au 7 Ag 6 units rotate by about 36° to form a staggered ( S ) configuration with D 5d symmetry ( S -Au 13 Ag 12 , Fig. 3d ). We note that, at the lower temperature (−10 °C), the Au 13 Ag 12 nanocluster prefers to adapt the configuration with a higher symmetry. The six chloride ligands—which bridge the two Au 7 Ag 6 units—serve as the “belt” to drive the rotamerization, Fig. 4 . In the E -Au 13 Ag 12 isomer, there are five Cl ligands with each being bonded with two silver atoms (d-mode). For the same isomer, there is also a Cl ligand that is bonded with four silver atoms (q-mode). In the S -Au 13 Ag 12 isomer, four Cl ligands are in the d-mode bonding, and two Cl ligands are each bonded with three silver atoms (t-mode). Fig. 4: Structures of E - and S -Au 13 Ag 12 isomers from the top view. Doubly (d), triply (t), and quadruply (q) binding patterns of six equatorial Cl ligands bridging the two icosahedra. Color codes: Au: yellow; Ag: blue; Cl: green. Full size image Reversible transformation between the E - and S - isomer The E -Au 13 Ag 12 and S -Au 13 Ag 12 isomers can be 100% selectively obtained at −10 and 25 °C, respectively. To test the reversibility of the isomeric transformation, we monitored the process by UV-vis absorption spectroscopy using the crystal sample of E -Au 13 Ag 12 nanoclusters as the starting material. We first studied the E -Au 13 Ag 12 nanocluster in a dichloromethane solution at 25 °C. The characteristic peak at 361 nm gradually decreased over time and simultaneously peaks at 330, 423, and 657 nm gradually increased. The peak at 418 nm also red-shifted to 510 nm during a period of 28 days, Fig. 5a . The 31 P NMR test of the sample gave a doublet-splitting peak centered at 57.36 ppm (see Supplementary Figs. 6 and 7 ). These results indicate that the E -Au 13 Ag 12 isomer slowly converts to the S -Au 13 Ag 12 isomer at 25 °C. We next studied the transformation of the as-obtained S -Au 13 Ag 12 isomer at −10 °C. The characteristic peaks at 330 and 657 nm disappeared after 42 days. Meanwhile, the peak at 361 nm increased and the peak at 510 nm blue-shifted to 418 nm, demonstrating that the S -Au 13 Ag 12 isomer transforms to the E -Au 13 Ag 12 counterpart (Fig. 5b ). This is further supported by 31 P NMR analysis, as the NMR peak appears at 54.80 ppm (see Supplementary Figs. 8 and 9 ). Of note, no byproduct was formed during the reversible transformation, evidenced by the ESI-MS tests (see Supplementary Figs. 10 and 11 ). These results imply that both isomers are stable, and the isomeric transformation process is reminiscent of typical phase transitions. Fig. 5: UV-vis spectral evolution for the isomeric transformation of the nanoclusters. 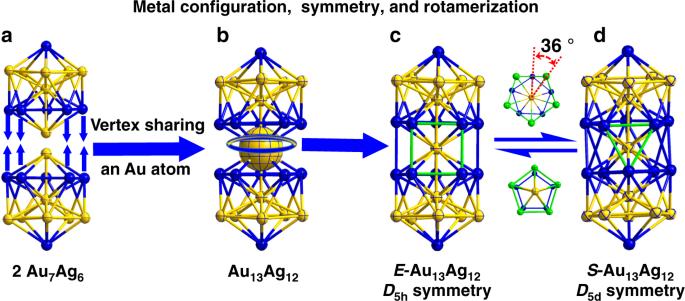Fig. 3: Configuration of the Au13Ag12nanocluster. a,bTwo icosahedral Au7Ag6units share one common vertex of Au to form the Au13Ag12nanocluster.cMetal configuration ofE-isomer.dMetal configuration ofS-isomer. Color code: Au: yellow; Ag: blue. Other atoms are omitted for clarity. a E -Au 13 Ag 12 conversion to S -Au 13 Ag 12 at 25 °C. b The as-obtained S -Au 13 Ag 12 conversion to E -Au 13 Ag 12 at −10 °C. Full size image Differential scanning calorimeter (DSC) method was used to investigate the isomeric transformation process and the corresponding enthalpy [28] . Starting from the S -Au 13 Ag 12 isomer, a negative peak centered at 79.6 °C was observed during the DSC test, which points to endothermicity of the isomeric transformation of the S -Au 13 Ag 12 to E -Au 13 Ag 12 (Fig. 6a ). Both UV-vis and 31 P NMR analyses indicate that the S -Au 13 Ag 12 isomer was partially converted to the E -Au 13 Ag 12 isomer (see Supplementary Figs. 12 and 13 ). Furthermore, thermogravimetric analysis (TGA) revealed that the removal of Cl ligands from the nanoclusters occur at 175 °C (weight loss of ~3.7 wt%, consistent with the expected value of 4.0 wt%), Fig. 6b . Subsequently, the phosphine ligands began to desorb at ~210 °C, consistent with the desorption temperature reported for the phosphine-protected Au nanocluster [28] , [29] . The TGA results indicate that the Au 13 Ag 12 nanoclusters are intact below 100 °C (see Supplementary Figs. 14 and 15 ); thus the observed endothermic process in the DSC analysis is solely associated with the isomeric transformation, rather than with any ligand loss. Fig. 6: Thermal analysis of the Au 13 Ag 12 nanoclusters. a DSC analysis for the conversion of the S -Au 13 Ag 12 to E -Au 13 Ag 12 under a N 2 atmosphere. b TGA test of the Au 13 Ag 12 nanoclusters under a N 2 atmosphere. Full size image Owning to the higher symmetry of the E -Au 13 Ag 12 ( D 5h ) than the S -Au 13 Ag 12 ( D 5d ), the nanocluster is a potential prototype of thermal molecular motor where Gibbs free energy serves as the driving force. In a previous work, Teo et al. [20] , [21] , [22] , [23] synthesized two isomers of Au 13 Ag 12 (PPh 3 ) 10 Br 8 nanoclusters; however, no isomeric rotamerization was observed, which can be attributed to the stronger Ag–Br bonds than Ag–Cl. Our study shows that employing the –Cl ligand, instead of –Br, leads to higher flexibility on Ag–halide bonds, which is essential and critical to achieve a more flexible cluster framework for the thermally responsive, reversible transformation between the E -Au 13 Ag 12 and S -Au 13 Ag 12 isomers. Such a Cl-ligand-induced rotary nanomotor is simulated based on the experimental structures (see Supplementary Movie 1 ). For practical applications, the temperature will serve as the driving force. In summary, two isomers of the biicosahedral [Au 13 Ag 12 (PPh 3 ) 10 Cl 8 ] + (counterion: [SbF 6 ] − ) nanocluster (i.e., S -Au 13 Ag 12 and E -Au 13 Ag 12 ) are discovered, and these two isomers are reversibly transformable by controlling the temperature. The metal configuration of the E -Au 13 Ag 12 isomer possesses a higher symmetry ( D 5h ) than that of the S -Au 13 Ag 12 isomer ( D 5d ) and is preferably formed at low temperature (−10 °C). As the temperature increases to 25 °C, the S -Au 13 Ag 12 isomer (lower symmetry) is exclusively formed. This study shows that the alloying and ligand engineering (i.e., Ag–halide bond) provide a rational strategy to make the framework of metal nanoclusters more flexible for achieving the conformational isomerism, which has the potential to be applied in designing intelligent molecular engines with Gibbs free energy as the driving force of the activity. Synthesis of Au 13 Ag 12 nanoclusters Au(I)PPh 3 Cl (25 mg, dissolved in 2 mL chloromethane/methanol with v : v = 1:1) was mixed with AgSbF 6 (17.2 mg, dissolved in 2 mL chloromethane/methanol with v : v = 1:1). The solution was stirred in dark and air atmosphere. Then the solution was cooled using an ice bath for 30 min, followed by dropwise addition of NaBH 4 solution (2 mg, dissolved in 4 mL ice cold methanol). The mixture was kept in the dark and stirred for another 24 h. Next, the temperature was increased slowly to 25 °C. The mixture was then dried via vacuum evaporation and washed with hexane (2 × 1 mL), leaving a black solid. Finally, the black solid was dissolved in 2 mL dichloromethane/methanol ( v : v = 1:1) and centrifuged at 10,000 rpm for 5 min. Red, plate-like crystals of E -Au 13 Ag 12 and S -Au 13 Ag 12 were obtained via slow diffusion of diethyl ether into the cluster solution over 6 weeks at −10 or 25 °C. 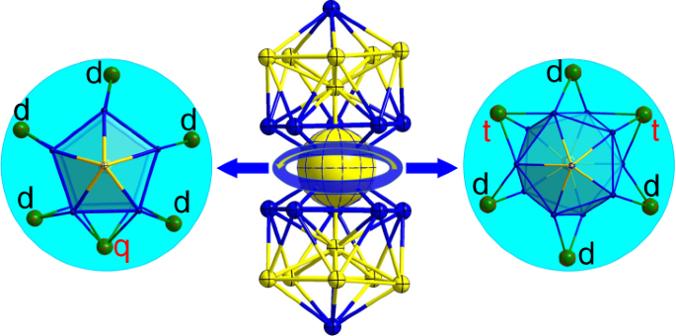Fig. 4: Structures ofE- andS-Au13Ag12isomers from the top view. Doubly (d), triply (t), and quadruply (q) binding patterns of six equatorial Cl ligands bridging the two icosahedra. Color codes: Au: yellow; Ag: blue; Cl: green. 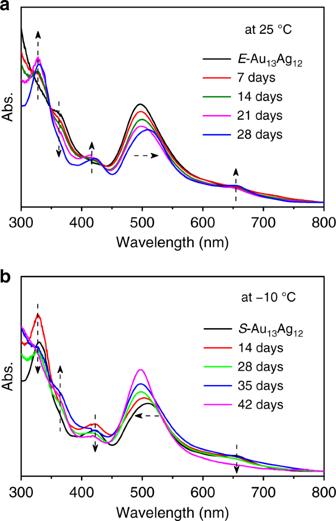Fig. 5: UV-vis spectral evolution for the isomeric transformation of the nanoclusters. aE-Au13Ag12conversion toS-Au13Ag12at 25 °C.bThe as-obtainedS-Au13Ag12conversion toE-Au13Ag12at −10 °C. 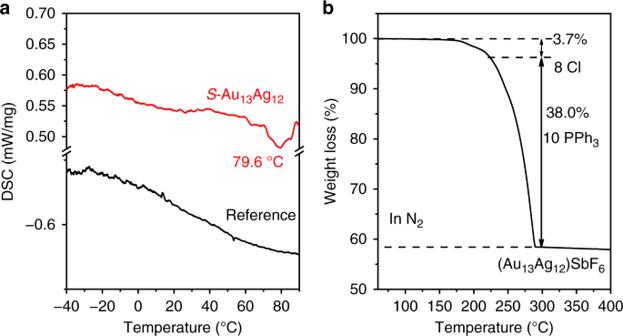Fig. 6: Thermal analysis of the Au13Ag12nanoclusters. aDSC analysis for the conversion of theS-Au13Ag12toE-Au13Ag12under a N2atmosphere.bTGA test of the Au13Ag12nanoclusters under a N2atmosphere. The yields are 26.0% for E -Au 13 Ag 12 and 34.9% for S -Au 13 Ag 12 based on the consumption of Ph 3 PAuCl.